Correspondence: DNA shape is insufficient to explain binding 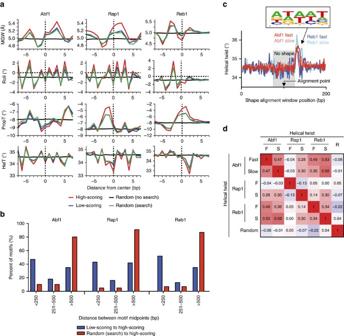Figure 1: Transcription factor motif-specific DNA shapes are not enriched at low scoring sites. (a) When the same search window is allowed to define the reference point for low-scoring (blue trace) and random (green trace) sites, the DNA shape patterns are indistinguishable from each other, unless no search window is employed (black trace). (b) The bp distance of each low-scoring site to the closest high-scoring site (blue bars) compared to the distance of each random site to the closest high-scoring site (red bars) for each factor. (c) Composite profiles of the aligned helical twist for Abf1 and Reb1 fast and slow sites. Other tested shape parameters behaved similarly (not shown). The frequency web logo is composed of all pentamers that possess an intrinsic helical twist larger than 35.5°. (d) Pearson correlations of the composite-aligned helical twist vectors for Abf1, Rap1 and Reb1 fast and slow, and random sites. The random sites for each factor were generated using the bedtools [6] random function, and then filtered to remove overlap with existing ChEC-seq peaks and overlap with each other. The underlying sequence in a 50 bp window around the random sites was then used to search for the best sequence match, using a normalized log-likelihood scoring metric [7] , to motifs for Reb1, Rap1 and Abf1 using consensus motifs from ScerTF [4] . The best match was then used to realign the random regions. DNA shape analysis [3] was performed on the existing high- and low-scoring ChEC-seq peaks along with the aligned and unaligned random regions. How to cite this article: Rossi, M. J. et al . Correspondence: DNA shape is insufficient to explain binding. Nat. Commun. 8 , 15643 doi: 10.1038/ncomms15643 (2017). Publisher’s note: Springer Nature remains neutral with regard to jurisdictional claims in published maps and institutional affiliations.